Erosion influences the seismicity of active thrust faults Assessing seismic hazards remains one of the most challenging scientific issues in Earth sciences. Deep tectonic processes are classically considered as the only persistent mechanism driving the stress loading of active faults over a seismic cycle. Here we show via a mechanical model that erosion also significantly influences the stress loading of thrust faults at the timescale of a seismic cycle. Indeed, erosion rates of about ~0.1–20 mm yr −1 , as documented in Taiwan and in other active compressional orogens, can raise the Coulomb stress by ~0.1–10 bar on the nearby thrust faults over the inter-seismic phase. Mass transfers induced by surface processes in general, during continuous or short-lived and intense events, represent a prominent mechanism for inter-seismic stress loading of faults near the surface. Such stresses are probably sufficient to trigger shallow seismicity or promote the rupture of deep continental earthquakes up to the surface. The evolution of the Earth’s topography is dictated by the interactions between tectonics, climate and surface processes (that is, erosion and sedimentation). Whether this evolution influences tectonic deformation during mountain building has been widely debated. It is now well accepted that surface evolution can drive the localization and intensity of tectonic deformation over geological times [1] , [2] , [3] (1–10 Myr). At intermediate time scales (10 kyr–1 Myr), erosion and the subsequent isostatic rebound can favour slip along specific fault planes [4] , [5] , [6] , [7] . However, the link between surface processes and the stress loading of faults during the seismic cycle (0.1–1 kyr), and in turn the associated deformation mechanisms, remains unsubstantiated. Faults represent the main mechanical discontinuities of the elastic–brittle Earth’s upper crust. They accommodate tectonic deformation by slipping, mostly during earthquakes [8] . These seismogenic faults are rooted down dip in viscous shear zones [8] , [9] , [10] . It is generally accepted that, during the inter-seismic phase (that is, before an earthquake), continuous viscous flow in these deep shear zones leads to the elastic stress loading of active faults closer to failure, and that during the co-seismic phase (that is, during an earthquake), failure and slip occur along the previously locked fault planes, followed by post-seismic stress relaxation [4] , [8] . Fault failure is commonly defined by the mean of the Coulomb stress change, ΔCFF=Δτ+μ ′· Δσ n , a function of the fault effective friction μ ′, the shear Δτ (positive in the direction of slip) and normal Δσ n (positive if the fault is unclamped) stress changes [8] , [11] . Earthquakes can be triggered by tectonic stresses, but also by Coulomb stresses due to episodic and short-lived events such as hydrologic [12] or snow loading [13] , nearby earthquakes [14] , [15] , [16] , [17] and slow-slip events [18] . Here, we show that surface processes significantly contribute to the Coulomb stress loading of thrust faults during the seismic cycle. To illustrate and then demonstrate our point, we consider a mountain range in Taiwan where the rates of erosion [19] and tectonic deformation [20] , [21] are extremely high and among the best-documented in the world. We then investigate how erosion influences the stress loading of thrust faults using a simple model for the seismic cycle. Coulomb stress changes induced by erosion in Taiwan Our first model quantifies the Coulomb stress change ΔCFF generated by erosional unloading, as constrained from fluvial suspended sediment load measured over the 30 yr before the 1999 M w 7.6 Chi–Chi earthquake in central Taiwan [19] ( Fig. 1 and Methods). The three dimensional (3D) velocity field v , strain rate and stress rate tensors induced by erosion are computed in an elastic half-space using a Boussinesq approach ( Fig. 1c and Methods). We use simplified geometries for active thrust faults located in the foothills of Taiwan [22] (for details, see Methods) and assume a dip angle α of 30°, a 15 km deep brittle–ductile transition [22] and an effective friction μ ′ of 0.5 to compute Coulomb stress changes per unit time (or loading rates) ΔCFF due to erosional unloading on these faults. We find a maximum value of ~4 × 10 −3 bar yr −1 for the Coulomb stress change ΔCFF induced by erosional unloading on the Liuchia fault system (number 8 on Fig. 1 ) in southwestern Taiwan. Despite a low topographic relief, this area has the highest erosion rates documented in Taiwan (up to 24 mm yr −1 ), which are proposed to be controlled locally by a low substrate strength, a high storminess and a high seismic moment release rate [19] . However, most of the thrust faults located in the foothills still display a significant ΔCFF of ~0.5 × 10 −3 bar yr −1 , including the Chelungpu fault (number 3) that ruptured during the Chi–Chi earthquake. Integrated over a seismic cycle duration [23] of ~500 yr, a ΔCFF of 0.5 to 4 × 10 −3 bar yr −1 due to erosional unloading gives a net Coulomb stress change of 0.25–2.0 bar. Similar values of Coulomb stress change are documented elsewhere to contribute significantly to the stress loading and dynamics of active faults [12] , [13] , [14] , [15] , [16] , [17] , [18] . This suggests that erosional unloading can significantly influence the short-term dynamics of faults. 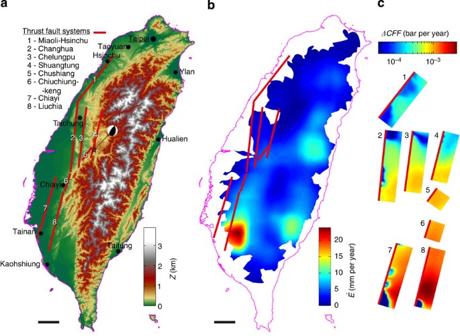Figure 1: Faults stress loading rates induced by erosion in the foothills of Taiwan. (a) Topography, simplified main thrust fault systems (red lines and numbers from 1–8) and location of the 1999Mw7.6 Chi–Chi earthquake epicenter (red star) that ruptured the Chelungpu fault (number 3). (b) Inter-seismic erosion rates before the Chi–Chi earthquake, as calculated from fluvial suspended sediment measurements with a 5-km grid resolution, smoothed at the catchment scale using a circular moving mean with 30-km diameter19. (c) Erosion induced Coulomb stress loading ratesΔCFFcalculated on the fault planes. The horizontal solid black lines represent scale bars of 50 km. Figure 1: Faults stress loading rates induced by erosion in the foothills of Taiwan. ( a ) Topography, simplified main thrust fault systems (red lines and numbers from 1–8) and location of the 1999 M w 7.6 Chi–Chi earthquake epicenter (red star) that ruptured the Chelungpu fault (number 3). ( b ) Inter-seismic erosion rates before the Chi–Chi earthquake, as calculated from fluvial suspended sediment measurements with a 5-km grid resolution, smoothed at the catchment scale using a circular moving mean with 30-km diameter [19] . ( c ) Erosion induced Coulomb stress loading rates ΔCFF calculated on the fault planes. The horizontal solid black lines represent scale bars of 50 km. Full size image Erosional unloading modifies the Coulomb stress change on a fault plane in two ways: (1) it decreases the normal stress and unclamps the fault, and (2) it increases the tangential stress ( Fig. 2a ). The increment of stress on a fault plane is proportional to the amount of erosion, but decreases with the square of the distance r between the fault plane and where erosion occurs ( Fig. 2b ). Therefore, the amplitude of erosional Coulomb stress loading on a fault is sensitive (1) to the effective friction μ ′, which modulates the effect of erosion on the normal stress, and (2) to the fault dip angle α , which decomposes the stresses into fault normal and tangential components and controls the distance of the fault plane to the surface. For instance, a higher effective friction μ ′ of 0.8 and a lower dip angle α of 15°, therefore, result in increasing the induced ΔCFF up to ~1 × 10 −2 bar yr −1 for the Liuchia fault system ( Fig. 2c ). In addition, the stresses modelled here are invariant with the Young modulus of the material, as we are considering a linear elastic material subjected to a surface pressure load (and not to a surface displacement). 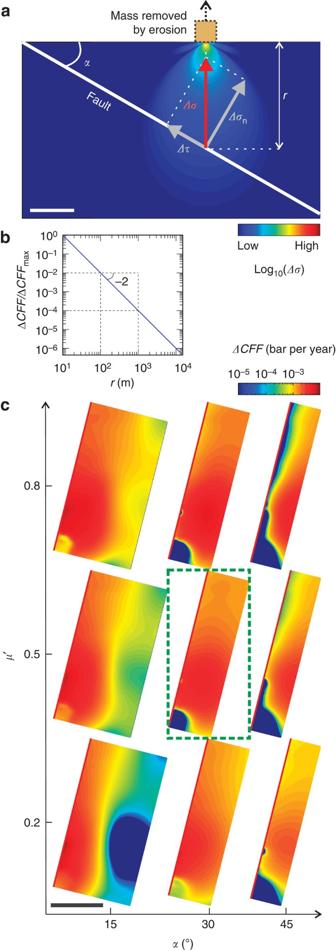Figure 2: Mechanism of Coulomb stress loading of a thrust fault by surface erosion. (a) Distribution of stress incrementΔσ(here purely illustrative) induced by a punctual erosion at the surface, increasing both the tangentialΔτ(driving effect) and the normal stressesΔσn(unclamping effect). The white solid line indicates a scale bar of 2.5 km. (b) The resulting fault Coulomb stress changeΔCFFdecreases with the square of the vertical distancerbetween the fault plane and where erosion occurs (assumingα=30° and 1 m of erosion). (c) Sensitivity ofΔCFFinduced by erosion to the fault dip angleαand effective frictionμ′, taking the Liuchia fault system as an example. The black solid line indicates a scale bar of 25 km. The model in the dashed green box is equivalent to the one inFig. 1andΔτandΔσnare reported inSupplementary Fig. 1. Figure 2: Mechanism of Coulomb stress loading of a thrust fault by surface erosion. ( a ) Distribution of stress increment Δσ (here purely illustrative) induced by a punctual erosion at the surface, increasing both the tangential Δτ (driving effect) and the normal stresses Δσ n (unclamping effect). The white solid line indicates a scale bar of 2.5 km. ( b ) The resulting fault Coulomb stress change ΔCFF decreases with the square of the vertical distance r between the fault plane and where erosion occurs (assuming α =30° and 1 m of erosion). ( c ) Sensitivity of ΔCFF induced by erosion to the fault dip angle α and effective friction μ ′, taking the Liuchia fault system as an example. The black solid line indicates a scale bar of 25 km. The model in the dashed green box is equivalent to the one in Fig. 1 and Δτ and Δσ n are reported in Supplementary Fig. 1 . Full size image Stresses induced by erosion during the seismic cycle The above computations consider inter-seismic erosion rates calculated from data acquired during the 30 yr preceding the Chi–Chi earthquake [19] . Even though its amplitude relative to co-seismic rock uplift is debated, co- and post-seismic erosional unloading represent a major contribution to erosion in seismic areas [24] , [25] , [26] , [27] . In mountain belts with hillslopes close to failure, co-seismic ground motion and acceleration can induce a significant amount of landslides [28] . The sediments produced by these landslides are then transported by rivers mainly during subsequent floods. This post-seismic landscape relaxation phase has a documented potential duration [25] , [26] of years to decades, one order of magnitude shorter than a complete seismic cycle. Therefore, the contribution of co- and post-seismic erosion to the stress loading of active faults also needs to be evaluated. To assess the relative contribution of inter-seismic erosion, co-/post-seismic erosion and tectonics to the Coulomb stress loading of faults, we develop a simple model of the seismic cycle that accounts for the effect of both erosion and tectonics ( Fig. 3 and Methods). We assume a steady-state landscape over the seismic cycle, that is, rock uplift rates are balanced by erosion rates Ė over this time scale. Because of the response-time of the geomorphic system to climate or tectonic perturbations and because of their stochastic properties [29] , this assumption is probably not valid in most settings. However, it offers a simple and self-consistent approach for modelling first-order surface processes during the seismic cycle. A Boussinesq approach is used to compute v , and , whereas the tectonic stresses and uplift (and therefore erosion) are calculated using dislocations embedded in an elastic half-space [30] . The effects of tectonic deformation during the inter- and co-seismic phases are accounted for by slip on a deep shear zone and on a shallow brittle fault, respectively [9] , [31] . This seismic cycle model is valid when considering a fault that is fully locked during the inter-seismic phase, as it is proposed for the thrust faults located in the western foothills of Taiwan [32] , [33] , [34] . 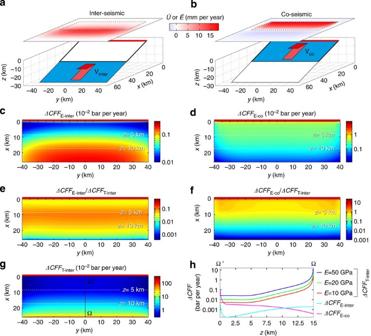Figure 3: Erosional versus tectonic driven Coulomb stress loading of faults during the seismic cycle. Model 3D geometry and modelled surface rock uplift rateduring the (a) inter- and (b) co-seismic phases averaged over the entire seismic cycle. The averaged tangential velocities of the shallow faultVcoand of the deep shear zoneVinterare equal to 40 mm yr−1. Erosional Coulomb stress loading rates of the fault obtained by equating erosion ratesĖto surface uplift ratesfor the (c) inter-seismicΔCFFE-interand (d) co-seismicΔCFFE-cophases. Ratios of (e) inter-seismic and (f) co-seismic erosional Coulomb stress loading rates over (g) the inter-seismic tectonic Coulomb stress loading rateΔCFFT-inter.ΔτandΔσnare reported inSupplementary Figure 2. (h) Spatial variation of Coulomb stresses along the fault plane (cross-section Ω-Ω′) considering different Young moduli (E=10, 20 and 50 GPa) that only influences the tectonics stresses and not the stresses induced by erosion. Figure 3: Erosional versus tectonic driven Coulomb stress loading of faults during the seismic cycle. Model 3D geometry and modelled surface rock uplift rate during the ( a ) inter- and ( b ) co-seismic phases averaged over the entire seismic cycle. The averaged tangential velocities of the shallow fault V co and of the deep shear zone V inter are equal to 40 mm yr −1 . Erosional Coulomb stress loading rates of the fault obtained by equating erosion rates Ė to surface uplift rates for the ( c ) inter-seismic ΔCFF E-inter and ( d ) co-seismic ΔCFF E-co phases. Ratios of ( e ) inter-seismic and ( f ) co-seismic erosional Coulomb stress loading rates over ( g ) the inter-seismic tectonic Coulomb stress loading rate ΔCFF T-inter . Δτ and Δσ n are reported in Supplementary Figure 2 . ( h ) Spatial variation of Coulomb stresses along the fault plane (cross-section Ω-Ω′) considering different Young moduli ( E =10, 20 and 50 GPa) that only influences the tectonics stresses and not the stresses induced by erosion. Full size image For comparison with faults in the foothills of Taiwan, we define a reference model with a fault trace length of 80 km and a dip angle of 30°, while keeping all the other mechanical properties identical. We also impose a slip velocity V inter of 40 mm yr −1 on the shear zone during the inter-seismic phase, and V co of 40 mm yr −1 on the associated brittle fault during the co-seismic phase. This model setup provides only a rough approximation of the seismic cycle at the scale of the whole western foothills of Taiwan. Indeed, deformation is partitioned between several active thrust faults in this area that are probably rooted down at depth into a single decollement with a total slip of ~40 mm yr −1 (refs 21 , 33 ). In addition, because our goal is to quantify the co- and post-seismic erosional unloading rates during the landscape relaxation phase following large earthquakes [25] , [26] , we compute co-seismic slip velocity averaged over the seismic cycle rather than co-seismic instantaneous displacement. Note that these two approaches are strictly equivalent in an elastic model. In our modelling, inter- and co-seismic rock uplift (and erosion) rates are similar and up to ~20 mm yr −1 ( Fig. 3 ). We assume no time modulation of inter- and co-seismic erosion and both modelled erosion rates are applied over the entire duration of one seismic cycle. Despite similar erosion rates, co-seismic erosional unloading induces fault Coulomb stress loading ΔCFF E-co of up to ~8 × 10 −2 bar yr −1 at very shallow depth (<1 km), which is about 30 times the maximum stress loading induced by inter-seismic erosion ΔCFF E-inter . Indeed, the maxima of co-seismic uplift of the surface (and erosion) occurs over the shallow portion of the fault, therefore at a shorter distance to the fault plane than the maxima of inter-seismic erosion ( Fig. 3 ). Despite a rapid decrease with depth, ΔCFF E-co is still greater than ~0.5 × 10 −2 bar yr −1 at a depth of 5 km. Coulomb stress loading ΔCFF E-inter induced by inter-seismic erosion displays two local maxima of ~0.3 × 10 −2 bar yr −1 , one located on the deeper part of the fault underneath the maximum of inter-seismic erosion, and the second one close to the fault tip owing to its proximity with the surface. We then compare fault Coulomb stress loading rates induced by erosion with those induced only by tectonics during the inter-seismic phase ΔCFF T-inter . In terms of amplitude, Coulomb stress loading rates due to tectonics are up to two or four orders of magnitude greater than those related to erosion, in particular for the deeper part of the fault. However, at shallower depths (<5 km), Coulomb stress loading rates due to co-seismic erosion and tectonics are of the same order of magnitude, and the ratio ΔCFF E-co / ΔCFF T-inter even reaches ~20 close to the surface ( Fig. 3 ). At the contrary, Coulomb stress loading rates associated with inter-seismic erosion, which is maximum on the deeper and shallower part of the fault, do not dominate tectonic stresses. The ratio ΔCFF E-inter / ΔCFF T-inter only reaches ~0.1 at intermediate depths (5–10 km) and ~0.6 close to the surface. Because the upper crust displays a very long stress relaxation time associated with high effective viscosities, these Coulomb stress changes induced by erosion can be accumulated over the time scale of a seismic cycle (~500 yr). On the other hand, increasing the Young modulus from the reference value (10 GPa) by a factor of 2 (20 GPa) or 5 (50 GPa) results in increasing the Coulomb stress change induced by tectonics ΔCFF T-inter by a factor of 2 or 5 and decreasing the ratios ΔCFF E-inter / ΔCFF T-inter and ΔCFF E-co /ΔCFF T-inter by the same factor ( Fig. 3h ). However, these results still demonstrate (1) that erosion can contribute significantly to thrust fault stress loading during the seismic cycle, and (2) that erosion can even be one of the dominant stress loading mechanisms for the shallower parts of thrust fault planes. Model sensitivity analysis To assess the sensitivity of our results to the model parameters, we design a set of models similar to the reference model, but with varying values of the effective friction μ ′ (0.1–0.9), the Young modulus E (10, 20 and 50 GPa) and the fault and shear zone dip angle α (15 to 45°). For the sake of simplicity, we keep the depth of the brittle–ductile transition at 15 km, which in turn implies that the surface area of the brittle fault increases when decreasing α . Using this modelling approach, erosion rates during the inter-seismic Ė inter and the co-seismic Ė co phases are only sensitive to α ( Fig. 4a,b ). Whereas Ė inter remains approximately constant around 13 mm yr −1 , Ė co increases from 11 to 22 mm yr −1 when α increases from 15–45°. 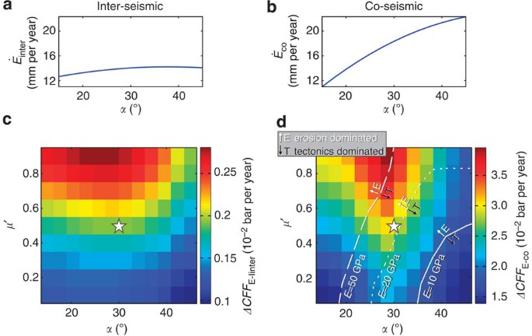Figure 4: Sensitivity of model results to the model parameters. Maximum surface erosion rates obtained during the (a) inter-seismicĖinterand the (b) co-seismicĖcoperiods as a function of the fault and shear zone dip angleα. Maximum fault Coulomb stresses induced by erosion during (c) inter-seismicΔCFFE-interand (d) co-seismicΔCFFE-coperiods, which are function of the dip angleαand of the effective frictionμ′, are shown with a plain colour map. White lines indicate the limits of tectonics (black arrow) versus erosion (white arrow) dominated Coulomb stresses in the model parameter space for varying values of the Young modulusE(10, 20 and 50 GPa). The reference model is represented by a white star. We consider that Coulomb stresses induced by erosion dominate tectonic stresses when at least one element of the fault is dominated by erosional stresses. For the inter-seismic erosion induced stresses, we here only consider the deep part of the fault. Figure 4: Sensitivity of model results to the model parameters. Maximum surface erosion rates obtained during the ( a ) inter-seismic Ė inter and the ( b ) co-seismic Ė co periods as a function of the fault and shear zone dip angle α . Maximum fault Coulomb stresses induced by erosion during ( c ) inter-seismic ΔCFF E-inter and ( d ) co-seismic ΔCFF E-co periods, which are function of the dip angle α and of the effective friction μ ′, are shown with a plain colour map. White lines indicate the limits of tectonics (black arrow) versus erosion (white arrow) dominated Coulomb stresses in the model parameter space for varying values of the Young modulus E (10, 20 and 50 GPa). The reference model is represented by a white star. We consider that Coulomb stresses induced by erosion dominate tectonic stresses when at least one element of the fault is dominated by erosional stresses. For the inter-seismic erosion induced stresses, we here only consider the deep part of the fault. Full size image The resulting Coulomb stresses ΔCFF E-inter and ΔCFF E-co on the fault plane are in turn sensitive to (1) the dip angle α , which controls both the distribution and amplitude of Ė inter and Ė co and the distance between the Earth surface and the fault plane, and (2) the effective friction μ ′ by amplifying the influence of normal stress on the Coulomb stress ( Fig. 4c,d ). The maximum values of ΔCFF E-inter and ΔCFF E-co obtained on the fault plane show similar distributions in the parameter space. ΔCFF E-inter is minimum (~1 × 10 −3 bar yr −1 ) for a low effective friction ( μ ′≤0.2) combined to a high or low dip angle (15° or 45°), whereas it increases when increasing μ ′ and reaches a maximum (~2.7 × 10 −3 bar yr −1 ) for α around 25°. ΔCFF E-co is minimum (~1.5 × 10 −2 bar yr −1 ) for a low effective friction ( μ ′≤0.2) combined to a high or low dip angle (15° or 45°), whereas it increases when increasing μ ′ and reaches a maximum of ~4 × 10 −2 bar yr −1 for α around 30°. Because the Coulomb stresses induced by tectonics ΔCFF T-inter are also sensitive to the Young modulus E , the ratios ΔCFF E-inter / ΔCFF T-inter and ΔCFF E-co /ΔCFF T-inter are in turn sensitive to α , μ ′ and E . Increasing the Young modulus from 10 to 20 or 50 GPa increases ΔCFF T-inter and decreases ΔCFF E-inter / ΔCFF T-inter and ΔCFF E-co /ΔCFF T-inter by a factor of 2 or 5, respectively. ΔCFF E-inter / ΔCFF T-inter remains lower than one only for all the models tested, independent of the Young modulus E . At the contrary, ΔCFF E-co /ΔCFF T-inter displays a large domain in the parameter space with values greater than one (that is, with at least one element of the fault plane dominated by stresses induced by erosion). For E =10 GPa, only models with low μ ′ (<0.5) and high α (>35°) are dominated by tectonic stresses ( ΔCFF E-co /ΔCFF T-inter <1), whereasile for E =50 GPa, most of the models with α greater than 20–30° are dominated by tectonic stresses. Therefore, Coulomb stresses induced by erosion during the seismic cycle represent a significant contribution to fault stress loading, even though their amplitude depends on the properties of the fault (dip angle, effective friction) and of the medium (Young modulus). Based on erosion data from Taiwan [19] , we have demonstrated that the elastic Coulomb stresses induced by erosion are of the order of ~0.5 × 10 −3 bar yr −1 on the thrust faults located in the western foothills and reach a maximum of ~4 × 10 −3 bar yr −1 on the Liuchia fault. These results are consistent with the outcomes from a simple model of the seismic cycle of a thrust fault that accounts for the effect of both erosion and tectonics, using fault properties and a slip velocity close to the ones inferred for Taiwan [20] , [21] , [22] . Coulomb stresses induced by inter-seismic ΔCFF E-inter and co-seismic ΔCFF E-co erosion and averaged over the duration of a seismic cycle (~500 yr) reach values of up to ~3 × 10 −3 bar yr −1 and ~8 × 10 −2 bar yr −1 , respectively. On the shallower part of thrust faults (<5 km deep), the ratio of the Coulomb stresses induced by co-seismic erosion ΔCFF E-co to the ones induced by tectonic loading ΔCFF T-inter is about equal to one for a Young modulus E =10 GPa (~0.2 for E =50 GPa) and even reach a maximum of ~20 closer to the surface (~4 for E =50 GPa). In addition, assuming that co-seismic erosion happens only during a period 10–100 times shorter [25] , [26] (~5–50 yr) than the complete seismic cycle [23] (~500 yr), ΔCFF E-CO increases up to 80 × 10 −1 to 8 bar yr −1 and the ratio ΔCFF E-co / ΔCFF T-inter to 10 or 100 for E =10 GPa (2–20 for E =50 GPa) during the first ~5–50 years following a large earthquake. Large earthquakes with a potential negative mass balance (that is, erosion greater than uplift), such as the Wenchuan earthquake [24] , [27] , could induce even higher rates of ΔCFF E-co than those predicted by a steady-state model. Our modelling approach imposes that co-seismic erosion is maximum close to the fault trace and above the shallower part of thrust faults ( Fig. 3 ). This result contrasts with most of the observed distribution of earthquake-triggered landslides, with a maximum of landslide density close to the epicentral area, and therefore generally above the deeper part of thrust faults [28] . Therefore, depending on the location of large earthquake hypocenters along the fault plane, our estimates for the contribution of co-seismic erosion to fault stress loading might likely be overestimated. However, our results emphasize that short-lived and intense erosional events associated with efficient sediment transport, such as typhoons, could suddenly increase the Coulomb stress of underlying faults. On longer time-scales, climatic changes or transition between fluvial- and glacial-dominated surface processes could also lead to high transient erosion rates and therefore to transient increases of the fault stress loading due to erosion [4] , [5] , [6] , [7] . The mechanism proposed in this study is limited neither to convergent settings nor to erosion only, as sediment deposition on the hanging wall of normal faults could also lead to a significant increase in Coulomb stress [5] . Moreover, some less active areas, such as intra-continental faults or old orogens still experience intense erosion and episodic seismic activity [6] , [7] . In the absence of major tectonic deformation, surface processes could significantly contribute to the stress loading of faults in these areas, even when considered independently of the stresses induced by isostatic rebound. In summary, our results demonstrate that surface processes represent a significant contribution to the Coulomb stress loading of faults during the seismic cycle. In terms of deformation, these additional stresses on the shallower part of fault planes can induce and trigger shallow earthquakes, as illustrated by the seismicity triggered by the large 2013 Bingham Canyon mine landslide [35] , or potentially favour the rupture of large deeper earthquakes up to the surface as, for instance, during the Chi–Chi earthquake [36] . This offers new perspectives on the mechanisms influencing stress transfers during the seismic cycle, as well as on seismic hazard assessment in areas experiencing rapid erosion. More generally, Coulomb stress loading of faults induced by surface processes over short time scales provides an additional positive feedback between climate, surface processes and tectonics. Seismic cycle model The deformation model computes the velocity field v , strain and stress rate tensors induced by surface erosion in a 3D elastic half-space based on the Boussinesq approximation [37] . With respect to this approximation, we assume that the model surface is horizontal ( Fig. 1 ). The effect of such assumption is here limited as the topography of the western foothills of Taiwan is globally <1 km. The model is discretized by cubic cells with a 100 m resolution, with a Young modulus of E =10 GPa, a Poison ratio of ν =0.25 and a rock density of ρ =2800, kg m −3 . Velocity, stresses and strain induced by tectonics are simulated by the mean of triangular dislocations [30] , [31] accounting for the slip (1) of a viscous deep shear zone during the inter-seismic phase and of (2) a frictional fault located in the shallow elastic–brittle crust during the co-seismic phase. The imposed averaged tangential velocities of the shear zone V inter and of the fault V co are both equal to 40 mm yr −1 . Coulomb stress changes are then computed by projecting the stresses due to surface processes and to tectonics on the fault plane that is discretized with a resolution of 100 m. The extent of fault planes and the dip angle data of the western foothills of Taiwan were simplified from ref. 22 . Each fault trace was simplified to a line segment that best reproduces the real fault trace geometry. Elastic Boussinesq model We here consider the displacements, stress and strain components generated by a point load F at the surface of a 3D semi-infinite elastic solid of coordinates x , y and z , with z being positive downward. Let’s define the distance to the point load of location ( x 0 , y 0 , z ), Δx = x − x 0 and Δy = y − y 0 . The elasticity of the model is described by the Lamé’s first λ and second parameters μ , which are related to the Young modulus E and the Poisson ratio ν by λ = Eν /((1+ ν )(1−2ν)) and μ = E /(2(1+ ν )) For z ≥0, the displacement components are [37] , [38] : Assuming infinitesimal deformation, the symmetric Cauchy strain tensor ε is then obtained by differentiating the displacement vector, . For an isotropic medium, the stress components are then given by the following equation, , where δ ij is the Kronecker delta. The six stress components are [37] , [38] : Because the model is linear and elastic, the total displacement, stress and strain components for any distribution of surface load are then computed by summation of the displacement, stress and strain components obtained for each individual point load. Taiwan erosion rates Erosion rates in Taiwan were calculated from fluvial suspended sediment load measured over the 30 yr before the 1999 M w 7.6 Chi–Chi earthquake, considering that the total fluvial sediment load contains 70% of suspended load [9] ( Fig. 1b ). Erosion rates were calculated assuming that suspended sediment load, measured at 130 gauging stations, represents 70% of the river total sediment load, and that catchment-wide erosion rates correspond to the total sediment load divided by sediment density and by drainage area [19] . The smoothed erosion map of Fig. 1 was then obtained using a circular averaging window with a radius of 30 km. The spatial resolution of the erosion map, even though coarse, still allows for resolving potential heterogeneities of ΔCFF induced by erosion between different faults and along each individual fault plane. How to cite this article : Steer, P. et al . Erosion influences the seismicity of active thrust faults. Nat. Commun. 5:5564 doi: 10.1038/ncomms6564 (2014).